Cytotoxicity of botulinum neurotoxins reveals a direct role of syntaxin 1 and SNAP-25 in neuron survival Botulinum neurotoxins (BoNTs) are the most potent toxins known to humans and are one of the six high-risk bioterrorism agents [1] , [2] . These toxins are produced by anaerobic Clostridium bacteria and include seven serotypes (BoNT/A–G). BoNTs are composed of a light chain (LC, ~50 kDa) and a heavy chain (~100 kDa) connected via a disulphide bond. The heavy chain contains a receptor-binding domain that targets neurons and a membrane translocation domain that translocates the LC into the cytosol. LCs act as proteases cleaving proteins required for synaptic vesicle exocytosis [1] , [2] . Specifically, BoNT/B, D, F and G cleave a vesicle protein synaptobrevin (Syb). BoNT/A, C and E cleave a peripheral plasma membrane protein SNAP-25. BoNT/C also cleaves a plasma membrane protein syntaxin 1 (Syx 1) ( Fig. 1a ). These three toxin substrates form the core complex essential for fusion of synaptic vesicle membranes to plasma membranes, known as SNARE proteins (soluble NSF attachment protein receptor) [3] . Cleavage of SNARE proteins blocks synaptic vesicle exocytosis and paralyzes humans and animals. 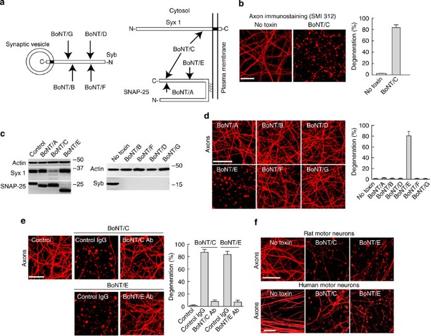Figure 1: BoNT/C and E can induce degeneration of cultured rodent and human neurons. (a) Schematic drawings of the cleavage sites on neuronal SNAREs for the seven BoNTs. BoNT/B, D, F and G cleave Syb. BoNT/A and E cleave SNAP-25. BoNT/C cleaves both Syx 1 and SNAP-25. (b) Cultured rat hippocampal neurons were exposed to BoNT/C (0.3 nM, 48 h). Axons were detected by immunostaining with an antibody specific for axonal neurofilament (SMI 312). Hippocampal neurons normally display continuous intact axons, whereas degenerated axons show severe beading and fragmentation. The percentage of degenerated axons was quantified (right panel), as described inSupplementary Fig. S1b. The same method was utilized to assay axon degeneration in all applicable figures. Cultured rat hippocampal neurons were used in all experiments, unless otherwise indicated in the figure legends. Scale bar, 20 μm. (c) Neurons were exposed to the seven BoNTs, respectively, for 12 h in media. Cell lysates were collected for immunoblot analysis detecting the indicated proteins. Actin served as the internal control for loading. Cleavage of SNAP-25 by BoNT/A, C and E generated fragments with smaller molecular weight. The Syx 1 fragment generated by BoNT/C was degraded within cells, resulting in multiple weak bands. Cleavage of Syb by BoNT/B, D, F and G resulted in loss of its immunoblot signals. (d) Neurons were exposed to the indicated six BoNTs for 48 h. BoNT/E, but not other toxins, induced axon degeneration. (e) Neurons were exposed to BoNT/C or BoNT/E that had been pre-incubated with control immunoglobulin G (IgG), a polyclonal anti-BoNT/C antibody (Ab, antibody, 1:200) or a polyclonal anti-BoNT/E antibody (1:200) as indicated. Cells were fixed 48 h later for assaying axon degeneration. (f) BoNT/C and E induced axon degeneration of both cultured rat motor neurons (upper panel) and human motor neurons derived from embryonic stem cells (lower panel). Error bars in all applicable panels represent s.e.m. Figure 1: BoNT/C and E can induce degeneration of cultured rodent and human neurons. ( a ) Schematic drawings of the cleavage sites on neuronal SNAREs for the seven BoNTs. BoNT/B, D, F and G cleave Syb. BoNT/A and E cleave SNAP-25. BoNT/C cleaves both Syx 1 and SNAP-25. ( b ) Cultured rat hippocampal neurons were exposed to BoNT/C (0.3 nM, 48 h). Axons were detected by immunostaining with an antibody specific for axonal neurofilament (SMI 312). Hippocampal neurons normally display continuous intact axons, whereas degenerated axons show severe beading and fragmentation. The percentage of degenerated axons was quantified (right panel), as described in Supplementary Fig. S1b . The same method was utilized to assay axon degeneration in all applicable figures. Cultured rat hippocampal neurons were used in all experiments, unless otherwise indicated in the figure legends. Scale bar, 20 μm. ( c ) Neurons were exposed to the seven BoNTs, respectively, for 12 h in media. Cell lysates were collected for immunoblot analysis detecting the indicated proteins. Actin served as the internal control for loading. Cleavage of SNAP-25 by BoNT/A, C and E generated fragments with smaller molecular weight. The Syx 1 fragment generated by BoNT/C was degraded within cells, resulting in multiple weak bands. Cleavage of Syb by BoNT/B, D, F and G resulted in loss of its immunoblot signals. ( d ) Neurons were exposed to the indicated six BoNTs for 48 h. BoNT/E, but not other toxins, induced axon degeneration. ( e ) Neurons were exposed to BoNT/C or BoNT/E that had been pre-incubated with control immunoglobulin G (IgG), a polyclonal anti-BoNT/C antibody (Ab, antibody, 1:200) or a polyclonal anti-BoNT/E antibody (1:200) as indicated. Cells were fixed 48 h later for assaying axon degeneration. ( f ) BoNT/C and E induced axon degeneration of both cultured rat motor neurons (upper panel) and human motor neurons derived from embryonic stem cells (lower panel). Error bars in all applicable panels represent s.e.m. Full size image BoNT’s ability to block synaptic vesicle exocytosis is also the basis for their medical applications: local injections of minute amounts of toxins can attenuate neuronal activities in targeted regions, which can be beneficial in many medical conditions. The unprecedented expansion of BoNTs in medical applications in recent years raises the pressing need to understand whether BoNTs can disrupt additional cellular functions beyond synaptic vesicle exocytosis. Indeed, it has been well documented that exposure to BoNT/C can cause degeneration of neurons in vitro and in vivo in mice [4] , [5] , [6] , [7] , [8] , [9] . If BoNTs only block synaptic vesicle exocytosis, they should not affect neuron viability, as synaptic vesicle exocytosis is not required for development and survival of neurons. For instance, tetanus neurotoxin, which blocks synaptic vesicle exocytosis by cleaving Syb, does not affect survival of cultured neurons [6] , [10] . Furthermore, lacking the presynaptic protein Munc13 completely abolishes synaptic vesicle exocytosis, yet Munc13-knockout (KO) mice develop normal brain structures, and neurons cultured from these mice grow normally in vitro [11] . Therefore, BoNT/C must disrupt additional functions in addition to blocking synaptic vesicle exocytosis. Why BoNT/C is toxic to neurons remains unknown, nor do we know whether any other BoNTs can induce death of neurons. Here we sought to address which BoNTs induce neurodegeneration, what toxin substrates are required for neuron survival and what cellular function via the action of BoNTs causes neurodegeneration. Our studies confirmed previous observations on BoNT/C cytotoxicity and revealed BoNT/E as the second BoNT to have cytotoxic effects on neurons. We established that cleavage of Syx 1 by BoNT/C and SNAP-25 by BoNT/E results in neurodegeneration. We further demonstrated that Syx 1/SNAP-25 act as SNARE proteins for supporting neuron survival, and the role of Syx 1/SNAP-25 can be substituted with any pairs of plasma membrane SNARE proteins. Finally, our data suggest that cytotoxicity is due to disruption of essential plasma membrane recycling processes, independent of blockage of synaptic vesicle exocytosis. BoNT/C and E induce degeneration of cultured neurons Using cultured rat hippocampal neurons as a model, we first developed an axon fragmentation assay to visualize and quantify BoNT/C-induced neuronal death ( Fig. 1b , Supplementary Fig. S1 ). Axon fragmentation is detected via immunostaining of axon-specific cytoskeleton protein neurofilament, and the percentage of fragmented axons is quantified using ImageJ software ( Fig. 1b , Supplementary Fig. S1b ). Consistent with previous characterizations by Berliocchi et al., [8] we found that sub-nanomolar levels of BoNT/C induced fragmentation of both axons and dendrites, and subsequent apoptosis of cell bodies, measured by multiple approaches ( Supplementary Fig. S1 ). Using the axon fragmentation assay, we first screened the other six BoNTs, which all can enter hippocampal neurons and cleave their target SNARE proteins ( Fig. 1c ). Of the six toxins screened, we found that BoNT/E induces axon degeneration and neuronal death ( Fig. 1d , Supplementary Fig. S2 ). BoNTs that cleave Syb (BoNT/B, D, F and G), as well as BoNT/A, do not affect axons and survival of neurons ( Fig. 1d ), demonstrating that blocking synaptic vesicle exocytosis is not the reason for neurodegeneration. Pre-incubation of BoNT/C and BoNT/E with their respective antibodies prevented axon degeneration ( Fig. 1e ), confirming that it is BoNT/C and E in toxin solutions that induce degeneration of neurons. In addition to hippocampal neurons, BoNT/C and E also induced degeneration of cultured rat motor neurons as well as human motor neurons derived from embryonic stem cells ( Fig. 1f ), demonstrating that these physiologically relevant target neurons are susceptible to cytotoxicity of BoNT/C and E. The other five BoNTs did not cause degeneration of rat or human motor neurons ( Supplementary Fig. S3 ). The BoNT/C and E protease domains induce death of neurons We next examined whether cytotoxicity of BoNT/C and E is due to the protease activity of their LCs ( Fig. 2a ). We expressed LCs of BoNT/C and E directly in neurons via lentiviral transduction. BoNT/A-LC was also assayed as a control. These LCs cleaved their target SNARE proteins in neurons ( Fig. 2b ). We found that both BoNT/C-LC and BoNT/E-LC induced axon degeneration and neuron death ( Fig. 2c ), whereas BoNT/A-LC did not affect neurons ( Fig. 2c ). 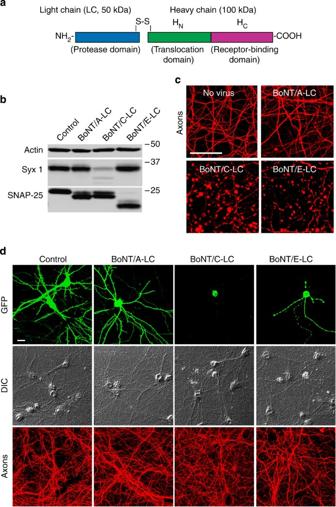Figure 2: The protease domains of BoNT/C and E induce cell-autonomous degeneration of neurons. (a) A schematic model of the three domain structures of BoNTs. (b) LCs of BoNT/A, C and E were expressed in neurons via lentiviral transduction. Cells were collected for immunoblot analysis 48 h later. LCs of BoNT/A, C and E cleaved their target SNARE proteins in neurons. (c) LCs of BoNT/A, C and E were expressed in neurons via lentiviral transduction. Cells were fixed for axon degeneration analysis 96 h later. LCs of BoNT/C and E, but not BoNT/A, induced axon degeneration. (d) High-density cultured hippocampal neurons were transfected with LCs of BoNT/A, C or E. To facilitate cell morphology analysis, neurons were co-transfected with a vector expressing GFP. Cells were fixed 48 h later and subjected to immunostaining analysis. Expression of BoNT/C-LC and E-LC resulted in degeneration of transfected neurons, without affecting neighbouring neurons. Scale bar, 20 μm. DIC, differential interference contrast. Figure 2: The protease domains of BoNT/C and E induce cell-autonomous degeneration of neurons. ( a ) A schematic model of the three domain structures of BoNTs. ( b ) LCs of BoNT/A, C and E were expressed in neurons via lentiviral transduction. Cells were collected for immunoblot analysis 48 h later. LCs of BoNT/A, C and E cleaved their target SNARE proteins in neurons. ( c ) LCs of BoNT/A, C and E were expressed in neurons via lentiviral transduction. Cells were fixed for axon degeneration analysis 96 h later. LCs of BoNT/C and E, but not BoNT/A, induced axon degeneration. ( d ) High-density cultured hippocampal neurons were transfected with LCs of BoNT/A, C or E. To facilitate cell morphology analysis, neurons were co-transfected with a vector expressing GFP. Cells were fixed 48 h later and subjected to immunostaining analysis. Expression of BoNT/C-LC and E-LC resulted in degeneration of transfected neurons, without affecting neighbouring neurons. Scale bar, 20 μm. DIC, differential interference contrast. Full size image We further found that expressing LCs of BoNT/C and E in only a few neurons by transfection resulted in degeneration of transfected neurons, suggesting that the cytotoxicity of BoNT/C and E is cell autonomous ( Fig. 2d ). The cytotoxicity is also likely specific to neurons, as LCs of BoNT/C and E did not affect survival of Neuro-2A cells, a neuroblastoma cell line that expresses Syx 1/SNAP-25, or primary glial cells ( Supplementary Fig. S4 ). Cleavage of Syx 1 by BoNT/C causes degeneration of neurons We next sought to identify the toxin substrate proteins whose cleavage leads to neurodegeneration. BoNT/C is known to cleave Syx 1 and SNAP-25 ( Fig. 1a ) [12] , [13] , [14] . Because BoNT/A cleaves one more residue from SNAP-25 than BoNT/C does ( Fig. 1a ), yet BoNT/A does not induce degeneration of neurons ( Figs 1d and 2c ), cleavage of SNAP-25 by BoNT/C is not the reason for its cytotoxicity. Therefore, we focused on Syx 1, which has two redundant isoforms, Syx 1A and 1B, in neurons. To test the role of Syx 1, we created toxin-resistant mutants, designated as Syx 1A/BoNT/C resistant (CR) and Syx 1B/CR, by changing four residues at the toxin cleavage site. The same mutations were used to create a mutant Syx 2 as a control, which is one of the four plasma membrane Syx family members (Syx 1–4) [3] . These CR mutants are resistant to BoNT/C in neurons ( Fig. 3a ). We found that Syx 1A/CR and Syx 1B/CR, but not Syx 2/CR, fully prevented BoNT/C-induced axon degeneration and neuron death ( Fig. 3b , Supplementary Fig. S5a,c ). Furthermore, expression of these CR mutants did not affect cleavage of endogenous Syx 1 and SNAP-25 by BoNT/C ( Fig. 3a , left panel), indicating that these toxin-resistant substrates did not protect neurons by deactivating BoNT/C. Instead, they likely replaced endogenous Syx 1. Together, these data demonstrate that cleavage of Syx 1 by BoNT/C causes neurodegeneration. 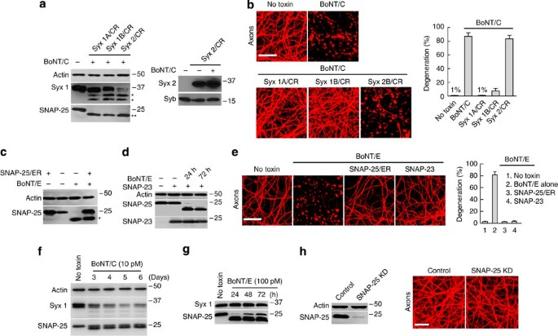Figure 3: Syx 1 and SNAP-25 are both required for neuron survival. (a) BoNT/CR mutants of Syx 1A, 1B and Syx 2 were expressed in neurons via lentiviral transduction. Cells were exposed to BoNT/C (0.3 nM, 12 h) and cell lysates were subjected to immunoblot analysis using antibodies for Syx 1 and SNAP-25 (left panel), or for Syx 2 (right panel). Syx 1A has a slightly lower molecular weight than Syx 1B. Cleavage of endogenous Syx 1 by BoNT/C generated multiple degraded fragments (left panel, marked by asterisks). Cleavage of SNAP-25 by BoNT/C generated a smaller fragment indicated by double asterisks. Actin and Syb served as loading controls. CR mutants are resistant to BoNT/C, and their expression did not affect cleavage of endogenous Syx 1 and SNAP-25 by BoNT/C. (b) Syx 1A/CR, 1B/CR and 2/CR were expressed in neurons. Neurons were exposed to BoNT/C and axon degeneration was analysed. (c) BoNT/E-resistant SNAP-25 mutant (SNAP-25/ER) was expressed in neurons. Neurons were exposed to BoNT/E and subjected to immunoblot analysis. Cleavage of SNAP-25 generated a smaller fragment marked by an asterisk. SNAP-25/ER is resistant to BoNT/E, and its expression did not affect cleavage of endogenous SNAP-25 by BoNT/E. (d) WT rat SNAP-23 was expressed in neurons via lentiviral transduction (+). Neurons were exposed to BoNT/E as indicated. WT SNAP-23 was not cleaved by nanomolar levels of BoNT/E in neurons. (e) SNAP-25/ER and SNAP-23 were expressed in neurons. Neurons were exposed to BoNT/E and axon degeneration was analysed. (f) Neurons were exposed to 10 pM BoNT/C for the indicated times. Cell lysates were collected and subjected to immunoblot analysis. (g) Neurons were exposed to 100 pM BoNT/E for the indicated times. Cell lysates were collected and subjected to immunoblot analysis. (h) SNAP-25 in neurons was knocked down via lentiviral-mediated shRNA. The KD efficiency was confirmed by immunoblot (left panel). KD SNAP-25 did not induce axon fragmentation (right panel), indicating that the residue levels of SNAP-25 are still sufficient to support neuron survival. Scale bar, 20 μm. Error bars in all panels represent s.e.m. Figure 3: Syx 1 and SNAP-25 are both required for neuron survival. ( a ) BoNT/CR mutants of Syx 1A, 1B and Syx 2 were expressed in neurons via lentiviral transduction. Cells were exposed to BoNT/C (0.3 nM, 12 h) and cell lysates were subjected to immunoblot analysis using antibodies for Syx 1 and SNAP-25 (left panel), or for Syx 2 (right panel). Syx 1A has a slightly lower molecular weight than Syx 1B. Cleavage of endogenous Syx 1 by BoNT/C generated multiple degraded fragments (left panel, marked by asterisks). Cleavage of SNAP-25 by BoNT/C generated a smaller fragment indicated by double asterisks. Actin and Syb served as loading controls. CR mutants are resistant to BoNT/C, and their expression did not affect cleavage of endogenous Syx 1 and SNAP-25 by BoNT/C. ( b ) Syx 1A/CR, 1B/CR and 2/CR were expressed in neurons. Neurons were exposed to BoNT/C and axon degeneration was analysed. ( c ) BoNT/E-resistant SNAP-25 mutant (SNAP-25/ER) was expressed in neurons. Neurons were exposed to BoNT/E and subjected to immunoblot analysis. Cleavage of SNAP-25 generated a smaller fragment marked by an asterisk. SNAP-25/ER is resistant to BoNT/E, and its expression did not affect cleavage of endogenous SNAP-25 by BoNT/E. ( d ) WT rat SNAP-23 was expressed in neurons via lentiviral transduction (+). Neurons were exposed to BoNT/E as indicated. WT SNAP-23 was not cleaved by nanomolar levels of BoNT/E in neurons. ( e ) SNAP-25/ER and SNAP-23 were expressed in neurons. Neurons were exposed to BoNT/E and axon degeneration was analysed. ( f ) Neurons were exposed to 10 pM BoNT/C for the indicated times. Cell lysates were collected and subjected to immunoblot analysis. ( g ) Neurons were exposed to 100 pM BoNT/E for the indicated times. Cell lysates were collected and subjected to immunoblot analysis. ( h ) SNAP-25 in neurons was knocked down via lentiviral-mediated shRNA. The KD efficiency was confirmed by immunoblot (left panel). KD SNAP-25 did not induce axon fragmentation (right panel), indicating that the residue levels of SNAP-25 are still sufficient to support neuron survival. Scale bar, 20 μm. Error bars in all panels represent s.e.m. Full size image Cleavage of SNAP-25 by BoNT/E causes degeneration of neurons BoNT/E is known to cleave SNAP-25 ( Fig. 1a ) [15] , [16] . We next created a BoNT/E-resistant SNAP-25 mutant, designated as SNAP-25/ER, by replacing four residues at the BoNT/E cleavage site ( Fig. 3c ). We also used SNAP-23 as a control, which is the other SNAP-25 family member. SNAP-23 is expressed in non-neuronal cells and developing neurons [17] , but its expression in mature hippocampal neurons is not detectable ( Fig. 3d , Supplementary Fig. S6a ). When expressed in neurons via lentiviral transduction, SNAP-23 was not cleaved by nanomolar levels of BoNT/E added to media ( Fig. 3d ), despite that it contains the toxin cleavage site and can be cleaved by high levels of BoNT/E-LC co-expressed in HEK293 cells ( Supplementary Fig. S6b ). These results indicate that SNAP-23 is not an effective substrate for BoNT/E in neurons. This finding allows us to test whether wild type (WT) SNAP-23 can prevent BoNT/E cytotoxicity. We found that both SNAP-25/ER and WT SNAP-23 fully prevented BoNT/E-induced axon degeneration and neuron death ( Fig. 3e , Supplementary Fig. S5b,c ), suggesting that SNAP-25 and SNAP-23 are functionally redundant in supporting neuron survival. Expression of these BoNT/E-resistant substrates did not affect cleavage of endogenous SNAP-25 by BoNT/E ( Fig. 3c ), indicating that SNAP-25/ER and SNAP-23 protected neurons by restoring essential cellular functions instead of deactivating BoNT/E. Because SNAP-23 is not expressed in mature neurons and it is not cleaved by nanomolar BoNT/E, we conclude that cleavage of endogenous SNAP-25 is the reason for BoNT/E-induced neurodegeneration. Consistent with our studies using active full-length toxins, co-transfecting toxin-resistant Syx 1A/CR with BoNT/C-LC, and SNAP-25/ER or SNAP-23 with BoNT/E-LC, respectively, prevented degeneration of transfected neurons ( Supplementary Fig. S7 ). In addition to hippocampal neurons, we found that Syx 1A/CR and SNAP-25/ER also rescued rat motor neurons and human motor neurons from BoNT/C and E, respectively ( Supplementary Fig. S8 ). As it has been argued whether inhibitory neurons express SNAP-25 (refs 18–20) [18] , [19] , [20] , we further examined the effect of BoNT/E on inhibitory neurons and found that BoNT/E can induce degeneration of both excitatory and inhibitory neurons ( Supplementary Fig. S9 ). These data support that SNAP-25 is expressed in inhibitory neurons. Cytotoxicity requires cleavage of nearly all Syx 1/SNAP-25 We next titrated BoNT/C and E to determine the minimal toxin concentrations that can induce degeneration of neurons. We found that BoNT/C at 10 pM and BoNT/E at 100 pM do not induce degeneration of cultured hippocampal neurons ( Supplementary Fig. S10 ). We then examined the residual Syx 1/SNAP-25 levels after neurons were exposed to BoNT/C and E at these concentrations. We found that BoNT/C at 10 pM eventually cleaved the majority of Syx 1 after 5 days ( Fig. 3f ). Syx 1 levels start to recover by day 6 ( Fig. 3f ), indicating that the toxin activity has started to decrease after 5 days. Because BoNT/C at 10 pM does not induce neurodegeneration, we conclude that the residue low level of Syx 1 at day 5 is still sufficient to support neuron survival. Similarly, we found that BoNT/E at 100 pM cleaved the majority of SNAP-25 by 24 h ( Fig. 3g ). Because BoNT/E has a shorter half-life than BoNT/C in neurons [21] , SNAP-25 starts to rise by 48 h after exposure to BoNT/E ( Fig. 3g ). Therefore, the residue low level of SNAP-25 at 24 h after exposure to BoNT/E is still sufficient to support neuron survival. To further confirm these conclusions, we used a different approach: knocking down (KD) endogenous SNAP-25 using lentiviral-mediated short hairpin RNA (shRNA) ( Fig. 3h ). The expression of SNAP-25 was reduced significantly ( Fig. 3h , left panel), yet we did not observe axon fragmentation and neurodegeneration ( Fig. 3h , right panel), suggesting that the residue level of SNAP-25 is still sufficient. Therefore, we conclude that only a minute percentage of endogenous Syx 1/SNAP-25 is needed to maintain neuron survival, and neurodegeneration only occurs when nearly all Syx 1/SNAP-25 are cleaved by toxins. BoNT/A-cleaved SNAP-25 does not tolerate additional mutations The finding that SNAP-25 is required for neuron survival raises a question: why does not BoNT/A induce neurodegeneration? The likely explanation is that BoNT/A only cleaves 9 amino acids, whereas BoNT/E cleaves 26 amino acids from the C terminus of SNAP-25 ( Fig. 4a ) [1] . To test this hypothesis directly, we constructed a SNAP-23 mutant that lacks the last nine amino acids. We used human SNAP-23 instead of SNAP-25 because human SNAP-23 is resistant to BoNT/E ( Supplementary Fig. S6c ). This allows us to avoid the inclusion of additional mutations at the BoNT/E cleavage site (an issue discussed further below). We found that this truncated SNAP-23 mutant can support neuron survival when endogenous SNAP-25 was abolished by BoNT/E ( Fig. 4b ). 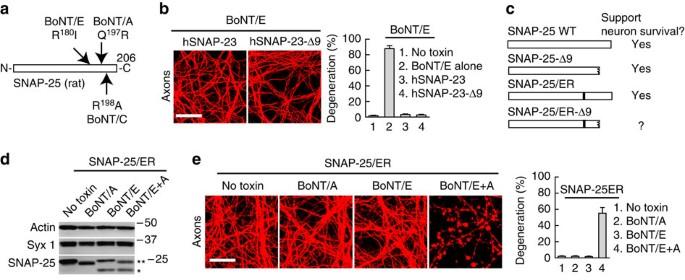Figure 4: SNAP-25 cleaved by BoNT/A has reduced capacity to tolerate additional mutations. (a) A schematic drawing of the cleavage sites for BoNT/A, C and E on rat SNAP-25. (b) Both full-length human SNAP-23 (hSNAP-23) and a truncation mutant lacking the last nine amino acids (hSNAP-23-Δ9) prevented axon degeneration in the presence of BoNT/E. (c) Schematic drawings showing mutants of SNAP-25 and their ability to support neuron survival. SNAP-25-Δ9 is the cleavage product generated by BoNT/A. The mutation site in SNAP-25/ER is marked in black. (d,e) SNAP-25/ER mutant was expressed in neurons via lentiviral transduction. Neurons were exposed to BoNT/A alone, BoNT/E alone or both BoNT/E and BoNT/A (BoNT/E+A). The single asterisk indicates the endogenous SNAP-25 cleaved by BoNT/E, whereas the double asterisk indicates the exogenous SNAP-25/ER cleaved by BoNT/A (d). When endogenous SNAP-25 was ablated by BoNT/E, cleavage of SNAP-25/ER by BoNT/A resulted in axon degeneration (e). Error bars in all panels represent s.e.m. Scale bar, 20 μm. Figure 4: SNAP-25 cleaved by BoNT/A has reduced capacity to tolerate additional mutations. ( a ) A schematic drawing of the cleavage sites for BoNT/A, C and E on rat SNAP-25. ( b ) Both full-length human SNAP-23 (hSNAP-23) and a truncation mutant lacking the last nine amino acids (hSNAP-23-Δ9) prevented axon degeneration in the presence of BoNT/E. ( c ) Schematic drawings showing mutants of SNAP-25 and their ability to support neuron survival. SNAP-25-Δ9 is the cleavage product generated by BoNT/A. The mutation site in SNAP-25/ER is marked in black. ( d , e ) SNAP-25/ER mutant was expressed in neurons via lentiviral transduction. Neurons were exposed to BoNT/A alone, BoNT/E alone or both BoNT/E and BoNT/A (BoNT/E+A). The single asterisk indicates the endogenous SNAP-25 cleaved by BoNT/E, whereas the double asterisk indicates the exogenous SNAP-25/ER cleaved by BoNT/A ( d ). When endogenous SNAP-25 was ablated by BoNT/E, cleavage of SNAP-25/ER by BoNT/A resulted in axon degeneration ( e ). Error bars in all panels represent s.e.m. Scale bar, 20 μm. Full size image The next question is whether BoNT/A cleavage attenuates the function of SNAP-25. One way to determine this is to introduce additional mutations to SNAP-25. If loss of the last nine amino acids weakens the function of SNAP-25, additional mutations that are tolerated in full-length SNAP-25 may cause loss of function in the truncated form because of additive effects. In fact, we already have a ‘perfect’ SNAP-25 mutant for this experiment: SNAP-25/ER mutant ( Fig. 3c ). This mutant can fully rescue neurons from BoNT/E, demonstrating that the mutations in it are tolerated in full-length SNAP-25. To determine whether SNAP-25/ER can afford to lose the last nine amino acids, we exposed neurons expressing SNAP-25/ER to both BoNT/E and BoNT/A. BoNT/E cleaved endogenous SNAP-25, virtually creating neurons that expressed only SNAP-25/ER. We found that cleavage of SNAP-25/ER by BoNT/A in these neurons induced death of neurons ( Fig. 4c–e ). These results demonstrate that SNAP-25 cleaved by BoNT/A has a reduced capacity to tolerate additional mutations. Syx 1/SNAP-25 act as SNARE proteins for neuron survival We next sought to determine whether Syx 1/SNAP-25 needs to form functional SNARE complexes for maintaining neuron survival. The pairing interfaces (layers −7 to +8) of Syx 1 and SNAP-25 in SNARE complexes have been well established [3] , [22] , [23] . We first examined two well-characterized point mutations in the SNARE interfaces: Syx 1 (A240V, V244A) and SNAP-25 (M71A). Both mutants lose the ability to mediate vesicle exocytosis [24] , [25] , [26] . When expressed in neurons via lentiviral transduction, these two mutants also failed to prevent toxin-induced degeneration of neurons, respectively ( Fig. 5a ). 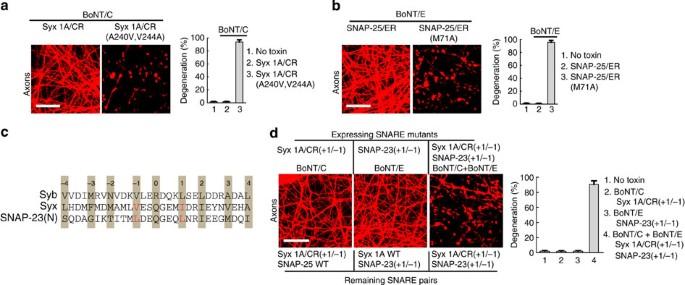Figure 5: Syx 1 and SNAP-25 act as SNARE proteins to support neuron survival. (a) Point mutations in Syx 1 (A240V, V244A) abolished the ability of Syx 1A/CR to prevent BoNT/C-induced neurodegeneration. (b) Point mutation (M71A) within the SNARE domain of SNAP-25 abolished the ability of SNAP-25/ER to prevent BoNT/E-induced degeneration. (c) The sequence alignment of the layer −4 to +4 interfaces in the middle portion of the SNARE complex containing Syx 1A, SNAP-23 and Syb. SNAP-23 contributes two helixes, with only the N-terminus helix shown in the alignment, which contains the targeted mutation sites. Layer −1 and 1 in Syx 1A/CR and SNAP-23 were highlighted in red and mutated to alanines (designated as Syx 1A/CR (+1/−1) and SNAP-23(+1/−1)). SNAP-23 was used to avoid additional mutations at the BoNT/E cleavage site. (d) Syx 1 A/CR(+1/−1) can prevent BoNT/C-induced axon degeneration. SNAP-23(+1/−1) can prevent BoNT/E-induced axon degeneration. However, a combination of Syx 1A/CR(+1/−1) and SNAP-23(+1/−1) failed to prevent axon degeneration in the presence of both BoNT/C and E. Error bars in all panels represent s.e.m. Scale bar, 20 μm. Figure 5: Syx 1 and SNAP-25 act as SNARE proteins to support neuron survival. ( a ) Point mutations in Syx 1 (A240V, V244A) abolished the ability of Syx 1A/CR to prevent BoNT/C-induced neurodegeneration. ( b ) Point mutation (M71A) within the SNARE domain of SNAP-25 abolished the ability of SNAP-25/ER to prevent BoNT/E-induced degeneration. ( c ) The sequence alignment of the layer −4 to +4 interfaces in the middle portion of the SNARE complex containing Syx 1A, SNAP-23 and Syb. SNAP-23 contributes two helixes, with only the N-terminus helix shown in the alignment, which contains the targeted mutation sites. Layer −1 and 1 in Syx 1A/CR and SNAP-23 were highlighted in red and mutated to alanines (designated as Syx 1A/CR (+1/−1) and SNAP-23(+1/−1)). SNAP-23 was used to avoid additional mutations at the BoNT/E cleavage site. ( d ) Syx 1 A/CR(+1/−1) can prevent BoNT/C-induced axon degeneration. SNAP-23(+1/−1) can prevent BoNT/E-induced axon degeneration. However, a combination of Syx 1A/CR(+1/−1) and SNAP-23(+1/−1) failed to prevent axon degeneration in the presence of both BoNT/C and E. Error bars in all panels represent s.e.m. Scale bar, 20 μm. Full size image We further examined whether there are additive effects between mutations in the same layer in Syx 1 and SNAP-25. To do so, we mutated residues at layers +1/−1 to alanines in both Syx 1A/CR and SNAP-23 ( Fig. 5c ). SNAP-23 was used to avoid additional mutations at the BoNT/E cleavage site. Syx 1A/CR(+1/−1) mutant prevented axon degeneration induced by BoNT/C, and SNAP-23(+1/−1) prevented axon degeneration induced by BoNT/E ( Fig. 5d ). However, when Syx 1A/CR(+1/−1) and SNAP-23(+1/−1) were expressed together, they failed to prevent axon degeneration in the presence of both BoNT/C and E ( Fig. 5d ). The likely explanation is that mutations at +1/−1 layers in Syx 1A and SNAP-23 are tolerated when pairing with endogenous WT partners, but they cannot form functional SNARE complexes with each other when endogenous WT SNAREs are eliminated with toxins. This additive effect demonstrates that Syx 1 and SNAP-25/23 need to pair with each other as SNARE proteins to support neuron survival. Other homologous SNARE pairs can support neuron survival In addition to mediating membrane fusion, Syx 1 and SNAP-25 have also been reported to interact with and regulate various ion channels [20] , [27] , [28] , [29] . The membrane fusion function of Syx 1/SNAP-25 is shared by other homologous plasma membrane SNARE proteins, namely Syx 2/3/4 for Syx 1 and SNAP-23 for SNAP-25 ( Fig. 6a ), whereas interactions with ion channels are often specific to Syx 1/SNAP-25. To further distinguish the role of Syx 1/SNAP-25 and to determine whether Syx 1 is the solo target responsible for BoNT/C-induced neuron death, we next examined whether Syx 1 can be substituted by Syx 2/3/4. Similar to SNAP-23, we found that Syx 2, 3 and 4 are not expressed at detectable levels in mature hippocampal neurons ( Fig. 6b–d ). When expressed exogenously via lentiviral transduction, Syx 2 and 3 were not cleaved by sub-nanomolar levels of BoNT/C ( Fig. 6b ), despite containing the BoNT/C cleavage sites. These findings indicate that Syx 2/3 are not effective substrates for BoNT/C in neurons. Syx 4 is known to be resistant to BoNT/C [13] ( Fig. 6d ). Despite being resistant to BoNT/C, we found that WT Syx 2/3/4 all failed to prevent BoNT/C-induced axon degeneration ( Fig. 6e ). 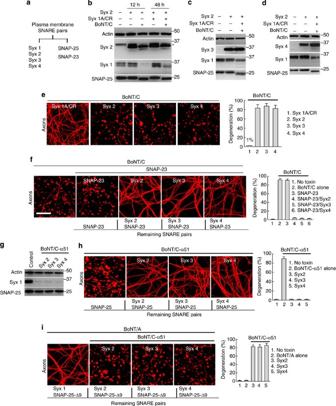Figure 6: Syx 1/SNAP-25 can be replaced by homologous SNARE proteins to support neuron survival. (a) A list of all known plasma membrane SNARE proteins. (b–d) WT Syx 2 (b), Syx 3 (c) and Syx 4 (d) were expressed in neurons via lentiviral transduction. Syx 1A/CR was co-expressed as indicated in each panel to prevent neuron death during the incubation with BoNT/C (0.3 nM, 48 h). Syx 2, 3 and 4 were detected using their specific antibodies. The Syx 2 antibody also cross-recognizes endogenous Syx 1, which is marked by an asterisk (b). Hippocampal neurons do not express detectable levels of endogenous Syx 2, 3 or 4. Exogenous WT Syx 2, 3 and 4 expressed via lentiviral transduction were not cleaved by 0.3 nM BoNT/C within 48 h in neurons. (e) WT Syx 2, 3, 4 and Syx 1A/CR were expressed in neurons. Neurons were exposed to BoNT/C, and axon degeneration was analysed. (f) Co-expressing exogenous SNAP-23 with Syx 2, 3 or 4 prevented axon degeneration induced by BoNT/C. Expressing SNAP-23 alone failed to prevent BoNT/C-induced axon degeneration. (g,h) A mutant BoNT/C-LC, BoNT/C-α51, which still cleaves Syx but loses the ability to cleave SNAP-25 (g), was co-expressed with Syx 2, 3 or 4 in neurons via lentiviral transduction. BoNT/C-α51 induced axon degeneration, which was prevented by Syx 2, 3 or 4 (h). (i) BoNT/C-α51 was co-expressed with Syx 2, 3 or 4 in neurons. Neurons were then exposed to BoNT/A. BoNT/A cleaved endogenous SNAP-25 and induced axon degeneration in neurons that express Syx 2/3/4. Scale bars, 20 μm. Error bars in all panels represent s.e.m. Figure 6: Syx 1/SNAP-25 can be replaced by homologous SNARE proteins to support neuron survival. ( a ) A list of all known plasma membrane SNARE proteins. ( b – d ) WT Syx 2 ( b ), Syx 3 ( c ) and Syx 4 ( d ) were expressed in neurons via lentiviral transduction. Syx 1A/CR was co-expressed as indicated in each panel to prevent neuron death during the incubation with BoNT/C (0.3 nM, 48 h). Syx 2, 3 and 4 were detected using their specific antibodies. The Syx 2 antibody also cross-recognizes endogenous Syx 1, which is marked by an asterisk ( b ). Hippocampal neurons do not express detectable levels of endogenous Syx 2, 3 or 4. Exogenous WT Syx 2, 3 and 4 expressed via lentiviral transduction were not cleaved by 0.3 nM BoNT/C within 48 h in neurons. ( e ) WT Syx 2, 3, 4 and Syx 1A/CR were expressed in neurons. Neurons were exposed to BoNT/C, and axon degeneration was analysed. ( f ) Co-expressing exogenous SNAP-23 with Syx 2, 3 or 4 prevented axon degeneration induced by BoNT/C. Expressing SNAP-23 alone failed to prevent BoNT/C-induced axon degeneration. ( g , h ) A mutant BoNT/C-LC, BoNT/C-α51, which still cleaves Syx but loses the ability to cleave SNAP-25 ( g ), was co-expressed with Syx 2, 3 or 4 in neurons via lentiviral transduction. BoNT/C-α51 induced axon degeneration, which was prevented by Syx 2, 3 or 4 ( h ). ( i ) BoNT/C-α51 was co-expressed with Syx 2, 3 or 4 in neurons. Neurons were then exposed to BoNT/A. BoNT/A cleaved endogenous SNAP-25 and induced axon degeneration in neurons that express Syx 2/3/4. Scale bars, 20 μm. Error bars in all panels represent s.e.m. Full size image We next considered the possibility that the reason Syx 2/3/4 failed to rescue neurons is because BoNT/C also cleaves SNAP-25 and truncates eight residues from its C terminus ( Fig. 4a ). We used two different approaches to address this issue. First, we circumvented it by expressing exogenous SNAP-23 in neurons, which is resistant to BoNT/C ( Supplementary Fig. S6b ) [30] . We found that co-expressing SNAP-23 with Syx 2/3/4 prevented BoNT/C-induced axon degeneration ( Fig. 6f ). Thus, the Syx 1/SNAP-25 pair can be replaced by exogenous pairs of Syx 2/3/4 with SNAP-23, which are plasma membrane SNARE pairs commonly found in non-neuronal cells. Second, we utilized a newly created mutant BoNT/C-LC (BoNT/C-α51) that only cleaves Syx 1, but loses the ability to cleave SNAP-25 ( Fig. 6g ) [31] . As expected, BoNT/C-α51 cleaved Syx 1 and still induced axon degeneration in neurons ( Fig. 6h ). Co-expressing exogenous Syx 2/3/4 in neurons prevented neurodegeneration induced by BoNT/C-α51, without the need to express SNAP-23 ( Fig. 6h ). These results demonstrate that Syx 2/3/4 can pair with full-length SNAP-25 to support neuron survival. Therefore, all possible combinations of known plasma membrane SNARE proteins, one from the Syx family, one from SNAP-25/23, can be used to support neuron survival. These findings demonstrate that the function of Syx 1/SNAP-25 for neuron survival depends on their intrinsic property as SNARE proteins for membrane fusion. SNAP-25 cleaved by BoNT/A cannot pair with Syx 2/3/4 As BoNT/A cleaves one more residue from SNAP-25 than BoNT/C, we expect that Syx 2/3/4 will not be able to pair with SNAP-25 cleaved by BoNT/A. To directly examine this possibility, we abolished Syx 1 in hippocampal neurons with BoNT/C-α51 while co-expressing Syx 2/3/4, virtually creating neurons that express Syx 2/3/4 instead of Syx 1. We found that BoNT/A readily induced axon degeneration in these neurons that rely on Syx 2/3/4 ( Fig. 6i ). Thus, the safety of BoNT/A depends on specific plasma membrane SNARE isoforms expressed in target neurons. Cytotoxicity is independent of synaptic vesicle exocytosis There are three major membrane fusion events at plasma membranes: (1) regulated vesicle exocytosis such as synaptic vesicle release; (2) constitutive exocytosis/secretion; and (3) exocytosis of plasma membrane recycling. We next examined which of these three routes is involved in toxin-induced neurodegeneration. We first further examined regulated synaptic vesicle exocytosis via sensitive electrophysiological recording of miniature excitatory postsynaptic currents (mEPSCs) ( Fig. 7a ). We confirmed that BoNT/A blocked synaptic vesicle exocytosis and abolished mEPSCs ( Fig. 7a ), yet it does not induce neurodegeneration ( Figs 1d and 2c ). Furthermore, Syx 1A/CR and SNAP-25/ER both failed to restore mEPSCs in neurons ( Fig. 7a ), despite their ability to prevent toxin-induced neurodegeneration. 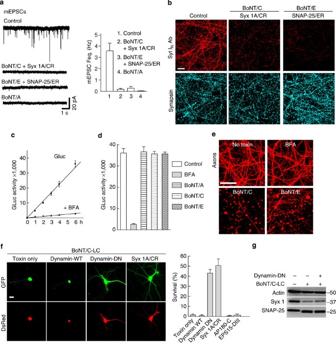Figure 7: Blocking endocytosis delays BoNT/C-LC-induced degeneration of neurons. (a) Neurons expressing Syx 1A/CR were exposed to BoNT/C, whereas neurons expressing SNAP-25/ER were exposed to BoNT/E. Neurons exposed to BoNT/A were examined as a control. Representative recordings (left panel) and frequencies (Feq. (Hz), right panel) of mEPSCs are shown. Syx 1A/CR and SNAP-25/ER both failed to restore mEPSC in the presence of toxins. (b) Neurons were exposed to BoNT/C or E as indicated for 6 h. Antibody uptake experiments were subsequently carried out using an antibody that recognizes the N-terminal domain of Syt I (Syt INAb) in the high K+solution. Syx 1A/CR and SNAP-25/ER failed to restore Syt INantibody uptake in neurons exposed to toxins. (c) A secreted Gluc assay was developed to monitor constitutive exocytosis in neurons. Gluc secreted into media showed a linear increase over time and was fully blocked by BFA. (d) Exposure to BoNT/A, C and E for 6 h did not reduce constitutive secretion of Gluc, whereas BFA completely blocked release of Gluc. (e) Neurons were exposed to BoNT/C, E and BFA for 36 h. The majority of neurons treated with BFA still remained intact, whereas BoNT/C and E have induced degeneration of neurons. (f) Co-transfection of a dominant-negative dynamin mutant (dynamin-DN, K44A), but not WT dynamin, with BoNT/C-LC delayed BoNT/C-LC-induced degeneration of neurons. Syx 1A/CR was used as a control. GFP was co-expressed in transfected cells to monitor neuron morphology. DsRed expression is driven by a separate promoter on the same vector as BoNT/C-LC, thus serving as a marker for BoNT/C-LC expression (lower panel). Percentages of survival cells 24 h after transfection were quantified in the right panel. Dominant-negative AP180 (AP180-C) and EPS15 (EPS15-DIII) that block clathrin-mediated endocytosis failed to affect BoNT/C-LC-induced degeneration of neurons in parallel assays (right panel). (g) Co-transfecting dynamin-DN (K44A) with BoNT/C-LC in Neuro-2A cells did not affect cleavage of Syx 1 and SNAP-25 by BoNT/C-LC. Error bars in all panels represent s.e.m. Scale bar, 20 μm. Figure 7: Blocking endocytosis delays BoNT/C-LC-induced degeneration of neurons. ( a ) Neurons expressing Syx 1A/CR were exposed to BoNT/C, whereas neurons expressing SNAP-25/ER were exposed to BoNT/E. Neurons exposed to BoNT/A were examined as a control. Representative recordings (left panel) and frequencies (Feq. (Hz), right panel) of mEPSCs are shown. Syx 1A/CR and SNAP-25/ER both failed to restore mEPSC in the presence of toxins. ( b ) Neurons were exposed to BoNT/C or E as indicated for 6 h. Antibody uptake experiments were subsequently carried out using an antibody that recognizes the N-terminal domain of Syt I (Syt I N Ab) in the high K + solution. Syx 1A/CR and SNAP-25/ER failed to restore Syt I N antibody uptake in neurons exposed to toxins. ( c ) A secreted Gluc assay was developed to monitor constitutive exocytosis in neurons. Gluc secreted into media showed a linear increase over time and was fully blocked by BFA. ( d ) Exposure to BoNT/A, C and E for 6 h did not reduce constitutive secretion of Gluc, whereas BFA completely blocked release of Gluc. ( e ) Neurons were exposed to BoNT/C, E and BFA for 36 h. The majority of neurons treated with BFA still remained intact, whereas BoNT/C and E have induced degeneration of neurons. ( f ) Co-transfection of a dominant-negative dynamin mutant (dynamin-DN, K44A), but not WT dynamin, with BoNT/C-LC delayed BoNT/C-LC-induced degeneration of neurons. Syx 1A/CR was used as a control. GFP was co-expressed in transfected cells to monitor neuron morphology. DsRed expression is driven by a separate promoter on the same vector as BoNT/C-LC, thus serving as a marker for BoNT/C-LC expression (lower panel). Percentages of survival cells 24 h after transfection were quantified in the right panel. Dominant-negative AP180 (AP180-C) and EPS15 (EPS15-DIII) that block clathrin-mediated endocytosis failed to affect BoNT/C-LC-induced degeneration of neurons in parallel assays (right panel). ( g ) Co-transfecting dynamin-DN (K44A) with BoNT/C-LC in Neuro-2A cells did not affect cleavage of Syx 1 and SNAP-25 by BoNT/C-LC. Error bars in all panels represent s.e.m. Scale bar, 20 μm. Full size image We also examined stimulated synaptic vesicle exocytosis by depolarizing neurons with high K + buffers and monitoring synaptic vesicle exocytosis using an antibody against the luminal domain of the major vesicle protein synaptotagmin I (Syt I, Syt I N Ab, Fig. 7b ). We found that Syx 1A/CR and SNAP-25/ER both failed to restore binding and uptake of Syt I N Ab in the presence of BoNT/C or E, respectively ( Fig. 7b ). Therefore, these toxin-resistant mutants separate two functions of Syx 1 and SNAP-25: they can support neuron survival, but cannot mediate synaptic vesicle exocytosis. BoNT/C and E do not affect constitutive exocytosis We next adopted a secreted Gaussia luciferase (Gluc) assay to test whether BoNT/C and E block constitutive exocytosis/secretion in neurons. Gluc possesses a natural secretory signal. Once expressed in neurons via lentiviral transduction, Gluc is released into media in a linear increase over time ( Fig. 7c ). Furthermore, Gluc release is fully blocked by brefeldin A (BFA), a potent blocker that disrupts secretory vesicle biogenesis ( Fig. 7c ), confirming that Gluc is released via constitutive secretion in neurons. By measuring Gluc levels in media, we found that BoNT/A, C and E did not affect Gluc secretion ( Fig. 7d ), indicating that these BoNTs do not disrupt constitutive exocytosis/secretion. Furthermore, blocking constitutive exocytosis/secretion using BFA did not induce axon fragmentation at the time point (36 h) when BoNT/C and E already induced severe axon fragmentation ( Fig. 7e ). Thus, constitutive exocytosis/secretion is not involved in toxin-induced neurodegeneration. Blocking endocytosis delays degeneration of neurons The third event is the exocytosis step during plasma membrane recycling processes. We reasoned that if cleavage of Syx 1 and SNAP-25 disrupts recycling processes by blocking the exocytosis step, blocking endocytosis may forcefully restore the balance at the plasma membrane temporarily. We first blocked clathrin-mediated endocytosis using dominant-negative AP180 (AP180-C) or EPS15 (EPS15-DIII) [32] , but both failed to affect toxin-induced degeneration of neurons ( Fig. 7f , Supplementary Fig. S11 ). We then blocked a broad range of endocytosis including both clathrin-dependent and clathrin-independent endocytosis using a dominant-negative dynamin (K44A) [32] . We found that dynamin (K44A) significantly delayed degeneration of neurons induced by co-expressed BoNT/C-LC ( Fig. 7f ). As dynamin (K44A) did not affect cleavage of Syx 1 by BoNT/C in cells ( Fig. 7g ), it is likely that blockage of endocytosis temporarily compensated the defects in exocytosis of plasma membrane recycling processes. Thus, these data suggest that BoNT/C and E induce neurodegeneration by disrupting exocytosis of essential dynamin-dependent recycling processes. Our studies expanded the previous observations on BoNT/C cytotoxicity and revealed BoNT/E as the second BoNT with cytotoxicity to neurons. We found that cytotoxicity only occurs when toxins can effectively cleave the majority of Syx 1 or SNAP-25 in neurons, indicating that only a small percentage of endogenous Syx 1/SNAP-25 is needed for supporting neuron survival. We estimated that the threshold concentrations for cytotoxicity to occur are >10 pM for BoNT/C and 100 pM for BoNT/E in cultured hippocampal neurons. These concentrations are far higher than the lethal dose in humans and animals, which is usually below femtomolar levels. Therefore, it is not likely that cytotoxicity has a significant role in pathogenesis of BoNT/C and E. On the other hand, BoNTs are used to target neurons locally via injections in therapeutic applications, and the same neurons are often exposed to BoNTs repeatedly over a long period of time. Because of this sustained toxin exposure, precautions should be taken in the use of BoNT/C and E as therapeutic toxins. Our studies establish that Syx 1/SNAP-25 are directly required for neuronal survival as the plasma membrane SNAREs for membrane recycling, independent of their well-known role for synaptic vesicle exocytosis. The specific cognate vesicle SNARE protein mediating essential membrane recycling processes remains to be identified. We expect it to be different from Syb, because BoNT/B, D, F and G that cleave Syb do not induce degeneration of neurons ( Fig. 1d ). The findings that exogenous SNAP-23 alone ( Fig. 6f ), or Syx 2/3/4 alone ( Fig. 6e ), both failed to prevent BoNT/C-induced degeneration of neurons, provide a functional readout, suggesting that there is no significant endogenous Syx 2/3/4 and SNAP-23 expression in mature hippocampal neurons. Thus, Syx 1/SNAP-25 are the predominant, if not the only, plasma membrane SNAREs and may act as promiscuous acceptors on plasma membranes in mature neurons. By limiting the expression to only Syx 1/SNAP-25, mature neurons may avoid potential interferences on neurotransmission from homologous SNARE proteins such as SNAP-23 that cannot support fast synaptic vesicle exocytosis [18] . This model is further supported by previous findings that Syx 1/SNAP-25 are broadly distributed along neuronal surfaces [33] , [34] , [35] . This model also predicts that Syx 1/SNAP-25 may act as the plasma membrane SNARE proteins for recycling of possibly all postsynaptic receptors and surface proteins in mature hippocampal neurons. This is supported by previous findings that SNAP-25 mediates protein kinase C-enhanced post-synaptic membrane insertion of NMDA ( N -methyl- D -aspartate) receptors and trafficking of kainate receptors [35] , [36] . Consistent with our conclusions that Syx 1/SNAP-25 are essential to neuron survival, it has been reported that hippocampal neurons cultured from SNAP-25 KO mice degenerate gradually in vitro [18] , [37] , which can be rescued by expressing SNAP-25, SNAP-23 or a SNAP-25 truncation lacking the nine residues at the C terminus [18] , [38] . Interestingly, SNAP-25 KO neurons can sustain the first few days of growth in vitro . This is likely because SNAP-23 is still expressed in developing neurons and its expression stops as neurons become mature ( Supplementary Fig. S6a ). The compensation from SNAP-23 also explains why the brain of SNAP-25 KO mice can develop normally until embryonic day 18 in vivo [37] , and stochastic expression of SNAP-23 may explain why a tiny percentage of SNAP-25 KO neurons (1.3%) can still survive for over 14 days in culture [18] . Syx 1 A/B double KO mice have not been generated because Syx 1 might be essential for embryonic viability [39] , [40] , [41] , [42] . Genetic studies in Drosophila have shown that Syx may mediate multiple membrane fusion events in different cells throughout development, including essential embryonic cellularization [40] , [41] , [42] . Furthermore, genetic mosaic analysis in Drosophila has demonstrated that lacking Syx causes cell lethality [43] . It is also interesting to note that lack of Munc-18, a Syx-binding protein essential for SNARE-mediated vesicle exocytosis in cells [44] , results in cell-autonomous degeneration of neurons [45] . Thus, it is likely that Munc-18 is also required for exocytosis in plasma membrane recycling processes. This is consistent with the hypothesis that both SNARE and SM (Sec1/Munc-18-like) proteins are required to form the minimal machinery for membrane fusion in cells [46] . Defects in CSPα, which is a co-chaperone for maintaining the SNAP-25 folding and facilitating SNARE complex assembly [47] , [48] , have been linked to neurodegenerative diseases [49] . In addition, α-synuclein may also act as a non-enzymatic chaperone to facilitate SNARE assembly [50] . Finally, changes of SNARE protein expression levels have been reported in Alzheimer’s disease and Huntington’s disease [51] , [52] , [53] . Our data establish a direct role for Syx 1/SNAP-25 in supporting neuron survival and suggest that disruption of house-keeping plasma membrane recycling processes might be a contributing factor in SNARE-related neurodegenerative processes. Antibodies and toxins Mouse monoclonal antibodies for Syx 1 (HPC-1), SNAP-25 (C171.2), Syb (C169.1) and Syt I (Syt I N Ab, Cl604.4) were generously provided by E. Chapman (Madison, WI). Rabbit polyclonal anti-BoNT/C and E were generated in E. Johnson’s lab (Madison, WI). The following antibodies were purchased from indicated vendors: mouse monoclonal antibodies for axonal neurofilament (SMI 312; Covance), actin (AC-15; Sigma-Aldrich), HA (16B12; Covance), NeuN (Millipore), ChAT (AB144P; Millipore) and GAD67 (1G10.2; Millipore); rabbit polyclonal antibodies against SNAP-23, Syx 2, Syx 4 (Synaptic Systems), synapsin and MAP-2 (Millipore); goat polyclonal antibody for Syx 3 (SC-47436; Santa Cruz Biotechnology). BoNT/A (Hall-A), BoNT/B (Okra), BoNT/C (Brazil), BoNT/D (D1873), BoNT/E (Alaska) and BoNT/F (Langeland) were purified in E. Johnson’s lab from the indicated strains. BoNT/G (G89) was purchased from Metabiologics (Madison, WI). The working concentrations in culture media are: BoNT/A (10 nM), BoNT/B (20 nM), BoNT/C (0.3 nM), BoNT/D (1 nM), BoNT/E (3 nM), BoNT/F (10 nM) and BoNT/G (20 nM), unless otherwise specified in the figure legends. cDNA and constructs The following cDNAs were generously provided by the indicated groups: human SNAP-23 (P. Roche, NIH) [17] , dynamin WT and K44A (S. Schmid, La Jolla, CA), AP180-C (L. Greene, NIH) and EPS15-DIII (A. Benmerah, France). The cDNA encoding LCs of BoNT/A (residues 1-448, M30196), C (residues 1-449, X53751), D (residues 1-445, AB012112) and E (residues 1-422, X62683) were synthesized by GenScript (New Brunswick, NJ) with codon optimized for eukaryotic cell expression. The cDNA encoding Gluc was purchased from NEB (Ipswich, MA). Syx 1A/CR, 1B/CR and 2/CR were generated by replacing residues at P2P1P1’P2’ of the BoNT/C cleavage site (KKAV in Syx 1A/1B, KKAI in Syx 2), with corresponding residues in Syx 5 (LIYF). SNAP-25/ER was generated by replacing residues at P3P2P1P1’ of the BoNT/E cleavage site (IDRI) in rat SNAP-25B with residues ‘NARE’. Other point mutations and deletions are specified in the figure legends. All constructs were sub-cloned into Lox-Syn-Syn lentiviral vectors, which contain two separate neuronal specific synapsin promoters. For constructs expressing toxin LCs, DsRed was co-expressed by the second synapsin promoter. For all other constructs, green fluorescent protein (GFP) was co-expressed. In Supplementary Figs. S4 and S6b , toxin LCs were sub-cloned into pcDNA3.1 vector with CMV promoters for overexpression in non-neuronal cells. Primary neuron and glial cell culture Dissociated rat hippocampal neurons were prepared from E18-19 embryos using a papain dissociation kit (Worthington Biochemical, NJ), as described previously [54] . Experiments were carried out using mature neurons after 14 days in vitro (DIV), unless otherwise indicated in the figure legends. Rat motor neurons were prepared from ventral spinal cords of E13 rats and dissociated with papain. Dissociated cells were loaded on the top of 7.05% NycoPrep (Accurate Chemical, NY) solutions and centrifuged (500 g , 20 min). Cells on the top of the solution were collected, re-suspended in a 3-ml Neurobasal medium and centrifuged (300 g , 5 min). Cell pellets were re-suspended and plated on poly- D -lysine-coated coverslips with a mono-layer of glial cells as described in detail below, at a density of 4 × 10 4 cells per well (24-well plate). Motor neurons were grown in a Neurobasal medium containing B27 supplement (Invitrogen) under 7% CO 2 . Glial cells were isolated from postnatal day 1 (P1) rat brain. Meninges were removed, cells were dissociated with trypsin (0.25%, 30 min) and cultured in the cell culture media (DMEM, 10% fetal bovine serum, 2 mM glutamine and 1% penicillin/streptomycin). After 7–9 days, cells were dissociated again with trypsin and plated onto coverslips at 20% confluence in the cell culture media. Arabinofuranosylcytosine was added to the media when the cells reached 100% confluence to inhibit cell proliferation. Transfection and lentiviral transduction Transfection of neurons was performed between DIV8 and DIV12 using the calcium phosphate method. HEK293 cells and a mouse neuroblastoma cell line Neuro-2A were transfected using Lipofectamine 2000 (Invitrogen). Lentiviral particles were generated using packaging vectors VSV-G and Δ8.9 as described previously [54] . Viruses were added to neurons at DIV5. Axon immunostaining and axonal degeneration quantification Culture neurons were fixed with 4% paraformaldehyde, permeabilized with 0.25% Triton X-100 and subjected to immunostaining using an antibody specific for axonal neurofilament (SMI 312, 1:1000). An Alexa-546 conjugated secondary antibody was usually utilized because many constructs co-express GFP. Images were collected using a confocal microscope (Leica TCS SP5; × 40 oil objective, Zoom 2). Quantification of axonal degeneration was carried out using ImageJ (NIH). Briefly, the axon immunostaining images were first converted into 8-bit black/white images and inverted, so axons display in black, then threshold was set to 180. The total axonal area was determined by measuring all pixels above threshold, including both intact and fragmented axons. Degenerated axons were detected using the Particle Analyzer module in ImageJ, by defining particle size between 10 and 500 pixels. This range of particle size covers the majority of observed beads and fragments of axons. The total area of particles divided by the total area of pixels is defined as the percentage of degenerated axons. Each experiment was repeated three times. Error bars in all figures represent s.e.m. Immunoblot analysis Cells were washed and lysed with RIPA buffer (50 mM Tris, 1% NP40, 150 mM NaCl, 0.5% sodium deoxycholate and 0.1% SDS) plus a protease inhibitor cocktail (Sigma-Aldrich). Lysates were centrifuged for 10 min at maximum speed using a microcentrifuge at 4 °C. Supernatants were subjected to SDS–polyacrylamide gel electrophoresis and immunoblot analysis using the enhanced chemiluminescence method (Pierce). Quantifying the survival rate of transfected neurons GFP was co-transfected with toxin LCs in neurons to assist cell morphology analysis. Twenty-four hours after transfection, GFP-positive neurons were counted as total transfected neurons using an epifluorescence microscope (Olympus IX 51; × 20 objective). Degenerated neurons were identified by their round cell bodies and fragmented neurites. Lentiviral-mediated shRNA KD of SNAP-25 SNAP-25 shRNA KD constructs were generated using the following primer: 5′-TGCTTAAATCCAGTGATGCTTTCAAGAGAAGCATCACTGGATTTAAGCTTTTTTC-3′, targeting the base pair 282–300 of rat SNAP-25. Annealed primers were cloned into the lentiviral vector pLL3.7 using Hpa I and Xho I sites. Expression of shRNA is driven by a U6 promoter, whereas a separate CMV promoter drives the expression of EGFP. Lentiviruses were added to neurons on DIV5. Experiments were carried out on DIV12–14. Constitutive secretion of Gluc Gluc was expressed in neurons via lentiviral transduction. The neurons were washed and 2 ml fresh media were added. Gluc secreted into the media was measured by taking 50 μl media and subjecting it to a luciferase activity assay using a kit following the manufacturer’s instructions (NEB, Ipswich, MA). To block constitutive secretion, cells were pre-treated with BFA (1 μg ml −1 ; Sigma-Aldrich) for 2 h before changing media and then further incubated in the presence of BFA for the indicated times. mEPSC recording Whole-cell patch-clamp recordings were performed at ambient temperature using a Multiclamp 700B amplifier (Molecular Devices). Cultured hippocampal neurons were bathed with an external solution containing (in mM) 126 NaCl, 2.5 KCl, 2.5 CaCl 2 , 1.2 MgCl 2 , 25 NaHCO 3 , 1.2 NaH 2 PO 4 and 11 D-glucose (pH 7.4, 300 mOsm). The patch electrodes were filled with (in mM): 130 K-gluconate, 8 NaCl, 10 Hepes, 0.4 EGTA, 5 QX-314 (lidocaine N-ethyl bromide), 2 Mg-ATP and 0.25 GTP-Tris (pH 7.25). The mEPSCs were recorded at the holding potential of −60 mV, with the presence of 1 μM tetrodotoxin blocking action potentials, 50 μM D-AP5 (D-2-amino-5-phosphonopentanoate) blocking NMDA receptors and 100 μM picrotoxin blocking GABA (γ-aminobutyric acid) receptors. Data were analysed with pClamp 10 (Molecular Devices) and Mini Analysis 6 (Synaptosoft). The threshold for detecting mEPSC events was set at 9 pA. Human motor neuron differentiation Human embryonic stem cells (lines H9, passages 19–35) were used to generate neuroectodermal cells. Motor neuron induction was carried out as previously described [55] . Briefly, human embryonic stem cell-derived neuroectodermal cells were treated with retinoic acid (0.1 μM; Sigma-Aldrich) for caudalization for 1 week in a chemically defined neural medium (NM: DMEM/F12, nonessential amino acids, 2 μg ml −1 heparin and the neural cell supplement N2 (Gibco)). The neuroepithelial clusters were isolated and suspended in the NM in the presence of both retinoic acid and purmorphamine (1 μM; Calbiochem). Purmorphamine was removed from the NM 1 week later. The formed progenitor spheres were subsequently cultured on glass coverslips coated with polyornithine and laminin (2–4 clusters per coverslip in a 24-well plate) in the presence of 0.5 ml NM, supplemented with brain-derived neurotrophic factor (10 ng ml −1 ; Peprotech), glial cell-derived neurotrophic factor (10 ng ml −1 ; R&D Systems), insulin-like growth factor 1 (10 ng ml −1 ; Peprotech), cyclic adenosine monophosphate (1 μM), ascorbic acid (200 ng ml −1 ; Innovative Cell Technology) and 50 nM retinoic acid. Cell media were changed every other day for long-term differentiation. How to cite this article: Peng, L. et al . Cytotoxicity of botulinum neurotoxins reveals a direct role of syntaxin 1 and SNAP-25 in neuron survival. Nat. Commun. 4:1472 doi: 10.1038/ncomms2462 (2013).